Towards enabling femtosecond helicity-dependent spectroscopy with high-harmonic sources Recent advances in high-harmonic generation gave rise to soft X-ray pulses with higher intensity, shorter duration and higher photon energy. One of the remaining shortages of this source is its restriction to linear polarization, since the yield of generation of elliptically polarized high harmonics has been low so far. We here show how this limitation is overcome by using a cross-polarized two-colour laser field. With this simple technique, we reach high degrees of ellipticity (up to 75%) with efficiencies similar to classically generated linearly polarized harmonics. To demonstrate these features and to prove the capacity of our source for applications, we measure the X-ray magnetic circular dichroism (XMCD) effect of nickel at the M 2,3 absorption edge around 67 eV. There results open up the way towards femtosecond time-resolved experiments using high harmonics exploiting the powerful element-sensitive XMCD effect and resolving the ultrafast magnetization dynamics of individual components in complex materials. High-harmonic generation in gas [1] results from the strong nonlinear polarization induced on a gas medium (most often a rare gas) by focusing of a linearly polarized laser field to an intensity of about 10 14 W cm −2 ( I ω ). Microscopically, every half optical cycle, electrons are snatched out of their parent atom, accelerated in the intense driving electric field, and then accelerated back to the atom when the electric field reverses. When recombining with the atom core, the electrons liberate their accumulated kinetic energy as an attosecond [2] burst of photons. This gives rise to the emission of a series of highly coherent odd harmonics spanning a wide range of the electromagnetic spectrum from the near ultraviolet to the soft X-rays. For years, the weak efficiency of this process has limited applications of this type of femtosecond light source but recent advances have allowed high harmonics to be used in photon-demanding applications. A second important limitation lies in the lack of circular polarization. As the high-harmonic beam polarization follows the atomic dipole direction, which is directly related to the driving laser polarization, one should expect to control the harmonic ellipticity by the driving laser ellipticity [3] , [4] , [5] . However, the recombination probability and consequently the harmonic generation efficiency drops dramatically with this latter [6] , [7] . Several methods were proposed to overcome this restriction [8] , [9] , [10] , [11] , [12] , [13] , [14] , [15] , [16] , but only three of them really show the production of high harmonics with elliptical polarization and non-negligible efficiency. The first possibility consists in generating harmonics in pre-aligned molecules [17] , [18] , [19] . In this approach, however, the measured ellipticity can hardly exceed 35% and only for harmonics corresponding to the low efficiency part of the generated spectrum. Alternatively, the linear polarization of the harmonics can be converted into circular polarization using a reflector phase shifter [20] . This technically challenging system reduces unfortunately the harmonic signal by one to two orders of magnitude depending on the degree of circular polarization required, and is limited to photon energies below ~70 eV. Finally, high harmonics were recently experimentally generated with controllable polarization using bichromatic elliptically polarized pump beams that interact with isotropic media [21] . All of the techniques require a relatively complex optical set-up, with several separated beams and/or an important number of optical components. None of these has allowed, up to now, to perform relevant applications at short wavelengths, demonstrating undoubtedly the high ellipticity and the important number of photons of their sources. In this letter, we show for the first time that one can achieve efficient generation of high harmonics at short wavelengths (here up to 70 eV), with a high degree of elliptical polarization (up to 75%), and in a compact and extremely simple system, using an orthogonally polarized two-colour ( ω +2 ω ) laser field. This scheme, involving only a frequency doubling crystal, was extensively investigated over the past years. In particular, it was established that harmonic pulses, containing both odd and even orders, can be generated with improved efficiency [22] , [23] , [24] , [25] , [26] compared with single-colour harmonic generation. The polarization of the harmonics, generated in such a specific case of orthogonally polarized ω and 2 ω laser fields in a centrally symmetric gas medium, was not measured so far and was expected to be linear [27] . The break of the temporal translation symmetry of the system (atom+fields) leading to the generation of elliptically polarized light can, however, be explained by taking into account non-zero projections of the orbital quantum number of the atoms states [28] . In addition, nonlinear processes inside the crystal, for instance a shift of the second harmonic frequency and possible ionization inside the gas medium may further break the symmetry. Polarimetry of the harmonic source Our experiment is carried out using a 1 kHz Ti:Sa laser system at ~800 nm ( ω ) delivering a few millijoules energy in 38-fs pulses (full width at half maximum) with linear polarization. The second harmonic (2 ω ) is generated by inserting a barium borate oxide (BBO) crystal into the laser path ( Fig. 1a ), both beams therefore overlap automatically inside the atomic gas medium. The 2 ω beam also has a linear polarization. With respect to the incident radiation, its polarization is turned by 90 degrees and it presents a phase shift of ~п/2 (see Methods). Due to dispersion effects inside the crystal (2 ω propagates faster than ω ), its thickness is restrained to a couple of micrometres to limit the temporal delay between the two pulse envelopes (Δ t , Fig. 1a ) and thus to preserve the high efficiency of the harmonic generation. The polarization of the harmonics, each order being well separated by a spectrometer, is determined using intensity measurements after an optical analyser set at different angles around the optical axis spanning a range of 200 degrees ( θ , Fig. 1b ). The angular dependence, following Malus’s law, is sinusoidal (see Methods) with a periodicity of 180 degrees ( Fig. 2a ). The amplitude of this oscillation is inversely proportional to the ellipticity and the angular position of the intensity maximum reflects the axis of the linear polarization. It is readily apparent that both odd and even harmonics have a varying degree of ellipticity. For example, the amplitude for the three consecutive harmonic orders 38th, 39th and 40th generated from ω +2 ω with a 100-μm-thick BBO crystal is much smaller than the amplitude of the linearly polarized 39th harmonic obtained from ω only. To quantify the ellipticity of each harmonic in two-colour configuration ( ε ω+2ω ), the intensity extrema of the sinusoidal oscillation ( I min and I max ), obtained using either ω +2 ω or ω only are inserted into equation (1) (see Methods). In this case, the very realistic assumption that harmonics generated using only a linear driving field ω are linearly polarized is made. 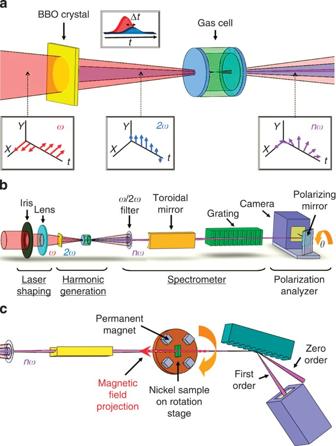Figure 1: Overview of the orthogonally polarized two-colour (ω-red,2ω-blue) high-harmonic (nω-violet) generation and XMCD experiment. (a) Generation of highly elliptically polarized high harmonics. The insets represent the polarizations ofω, of 2ωand of the harmonics (nωwithnas an integer); the approximate temporal disposition of theωand 2ωpulse envelops with Δtthe temporal delay between them. (b) Side view of the polarization measurement set-up.θis the analyzer angle. (c) Top view of the XMCD measurement set-up. Figure 1: Overview of the orthogonally polarized two-colour ( ω -red, 2ω -blue) high-harmonic ( nω -violet) generation and XMCD experiment. ( a ) Generation of highly elliptically polarized high harmonics. The insets represent the polarizations of ω , of 2 ω and of the harmonics ( nω with n as an integer); the approximate temporal disposition of the ω and 2 ω pulse envelops with Δ t the temporal delay between them. ( b ) Side view of the polarization measurement set-up. θ is the analyzer angle. ( c ) Top view of the XMCD measurement set-up. 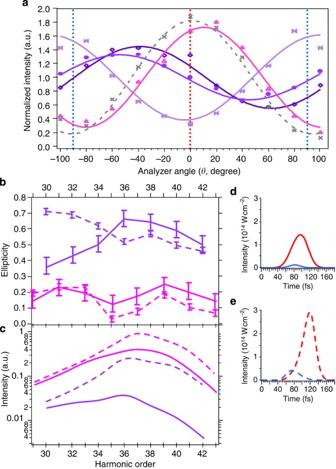Figure 2: Measurement of the ellipticity of the harmonics generated in orthogonally polarized two-colour configuration. (a) High-harmonic intensity measured as a function of the analyser angle (θ). The dotted lines indicate the polarization axis ofω(red) and 2ω(blue). The different markers correspond to the following harmonic numbers: 30th (bowtie), 38th (plain circle), 39th (triangle), 40th (diamond) and 39th fromωonly (cross) for direct comparison. Sinusoidal fits are provided (lines). (b,c) Measured ellipticity and intensity as a function of the harmonic orders: odd (pink) and even (violet). A 100-μm-thick BBO crystal case (plain line) withIω~1.5 × 1014W cm−2,I2ω~1.3 × 1013W cm−2and Δt=14 fs. A 250-μm-thick BBO crystal case (dashed line) withIω~3 × 1014W cm−2,I2ω~0.4 × 1014W cm−2and Δt=42 fs. (d,e) Temporal envelops ofω(red) and 2ω(blue) pulses, calculated by SNLO software, for respectively 100-μm (plain line) and 250-μm (dashed line)-thick BBO crystal. Full size image Figure 2: Measurement of the ellipticity of the harmonics generated in orthogonally polarized two-colour configuration. ( a ) High-harmonic intensity measured as a function of the analyser angle ( θ ). The dotted lines indicate the polarization axis of ω (red) and 2 ω (blue). The different markers correspond to the following harmonic numbers: 30th (bowtie), 38th (plain circle), 39th (triangle), 40th (diamond) and 39th from ω only (cross) for direct comparison. Sinusoidal fits are provided (lines). ( b , c ) Measured ellipticity and intensity as a function of the harmonic orders: odd (pink) and even (violet). A 100-μm-thick BBO crystal case (plain line) with I ω ~1.5 × 10 14 W cm −2 , I 2ω ~1.3 × 10 13 W cm −2 and Δ t =14 fs. A 250-μm-thick BBO crystal case (dashed line) with I ω ~3 × 10 14 W cm −2 , I 2ω ~0.4 × 10 14 W cm −2 and Δ t =42 fs. ( d , e ) Temporal envelops of ω (red) and 2 ω (blue) pulses, calculated by SNLO software, for respectively 100-μm (plain line) and 250-μm (dashed line)-thick BBO crystal. Full size image It has to be noted that the ellipticity values derived below are upper limits as our experimental procedure (analyser scans) cannot differentiate unpolarized light from elliptically polarized light [4] , [18] . While less than 20% ellipticity is reached for odd harmonics, above 40% is achieved for all even orders ( Fig. 2b ). An ellipticity as high as 65% is found for the 36th and 38th harmonic orders. We note that these harmonics also exhibit the highest intensity of the even orders ( Fig. 2c ). These observations suggest that while all harmonic orders are generated by a combination of both fields ( ω +2 ω ), their respective contributions vary with harmonic parity and order. Indeed, a higher degree of ellipticity for even orders implies a more significant impact of the 2 ω field compared to odd orders. Furthermore, higher orders, for which ellipticity is weaker, arise from higher intensities of the generation field, which here are reached at the rear part of the ω +2 ω pulse where the 2 ω field is smaller ( Fig. 2d ). To explore the possibility of reaching a higher degree of ellipticity for odd harmonics, a 250-μm-thick BBO crystal was used to increase the 2 ω generation efficiency and as a consequence the 2 ω intensity ( I 2ω ). A shift of the ellipticity peak to lower orders is observed. For the 38th harmonic, the ellipticity is reduced slightly to 55% ( Fig. 2b ) but the intensity is one order of magnitude higher ( Fig. 2c ). One also notes that the degree of ellipticity of the odd orders remains weak. These observations are consistent with a decrease of the interaction between the ω and 2 ω pulses (high Δ t ) due to the thicker BBO crystal ( Fig. 2e ). The solution is to keep the BBO thickness to the initial value (100 μm), ensuring a good temporal overlap, and to improve the second harmonic generation efficiency by increasing significantly the laser fluence on the BBO crystal. With higher I ω and I 2 ω and higher I 2 ω /I ω , one can then expect to reach much higher harmonic orders and higher ellipticity for odd orders. X-ray magnetic circular dichroism at nickel M 2,3 edge (67 eV) To definitively demonstrate the suitability of our technique for the generation of elliptically polarized harmonics and its maturity for applications, we directly measured, with this higher laser intensities configuration, the X-ray magnetic circular dichroism (XMCD) of a thin nickel film at the M 2,3 edge, which is located at ~67 eV. The XMCD effect is inherently only sensitive to elliptical light. 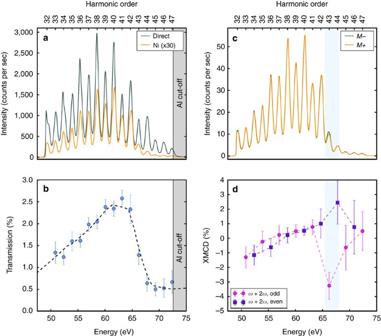Figure 3: Study of the XMCD effect at the Nickel M2,3edge using harmonics generated in orthogonally polarized two-colour configuration. A 100-μm-thick BBO crystal yieldingIω~4 × 1014W cm−2,I2ω~0.5 × 1014W cm−2and Δt=14 fs. (a) Transmission spectrum of harmonics through a Ni thin film (orange plain line) and reference harmonics spectrum (dark grey plain line). (b) Deduced experimental transmission of the Ni sample (blue circles). Calculated transmission (black dashed line) based on sample properties (see Methods). (c) Spectra of high harmonics transmitted through the Ni sample and obtained for the two magnetization directions (M+and M−). (d) Measured XMCD strength (odd orders in pink colour and even orders in violet colour). Details on the derivation of the XMCD signal are given in the Methods section. Incandd, the blue zone represents the known photon energy range of the XMCD effect at the Ni M2,3edge26. Figure 3a shows the harmonic spectra recorded with and without the Ni film. One notices a shift of harmonic yield toward higher orders. Also, even orders have now a slightly higher intensity than the adjacent odd orders. From these two spectra, we determine the transmission of the Ni film, which can be fitted easily by its theoretical transmission ( Fig. 3b ). Harmonic spectra recorded for opposite magnetization directions of the Ni film ( Fig. 3c and Methods Section) exhibit a different absorption for the 43rd harmonic, which is in resonance with the magnetically dichroic Ni M 2,3 absorption resonance. The presence of a magnetic dichroism thus indicates that the 43rd harmonic exhibits a significant degree of circular polarization. This observation is further evidenced by plotting the XMCD measurement (see Methods Section) as a function of harmonic order ( Fig. 3d ). One notes that the 43rd and 44th harmonics present a dichroism signal, which deviates clearly from the background and which is in line with the known photon energy range of the XMCD of the Ni M 2,3 edge [29] . In addition, the observed dichroism changes its sign for these two harmonics, while the Ni M 2,3 XMCD in absorption does not in the corresponding 65–69 eV range. This indicates that the two subsequent harmonics have an opposite helicity, an observation which has been predicted numerically [12] . Figure 3: Study of the XMCD effect at the Nickel M 2,3 edge using harmonics generated in orthogonally polarized two-colour configuration. A 100-μm-thick BBO crystal yielding I ω ~4 × 10 14 W cm −2 , I 2ω ~0.5 × 10 14 W cm −2 and Δ t =14 fs. ( a ) Transmission spectrum of harmonics through a Ni thin film (orange plain line) and reference harmonics spectrum (dark grey plain line). ( b ) Deduced experimental transmission of the Ni sample (blue circles). Calculated transmission (black dashed line) based on sample properties (see Methods). ( c ) Spectra of high harmonics transmitted through the Ni sample and obtained for the two magnetization directions (M + and M − ). ( d ) Measured XMCD strength (odd orders in pink colour and even orders in violet colour). Details on the derivation of the XMCD signal are given in the Methods section. In c and d , the blue zone represents the known photon energy range of the XMCD effect at the Ni M 2,3 edge [26] . Full size image We demonstrated that high harmonics with a high degree of ellipticity can be generated efficiently up to a photon energy of 70 eV using a simple and compact system. This enables the realization of XMCD measurement with femtosecond time resolution, a powerful technique, which has so far been only possible at femtoslicing facilities [30] or at X-ray free-electron lasers [31] , while a very limited number exists worldwide. In this regard, our extremely simple geometry opens up great opportunities for polarization-dependent spectroscopy techniques with table-top sources. Above all, with its natural femtosecond resolution, pump-probe jitter-free experiments to follow in real time the dynamics of ultrafast processes [32] are now possible. For example, nanoscale imaging of magnetic domains or chiral domains in biological systems using holographic techniques could be considered. Elliptically polarized harmonics could also be used as a seed for plasma X-ray amplifiers leading to very intense pulses of elliptically polarized soft X-rays. Finally, the potential of our technique for applications requiring higher photon energies is very strong since the process depends neither on the driving laser wavelength nor on the gas type, allowing it to be used with advanced high-harmonic generation schemes in any spectral range [33] . Harmonic generation in gas Harmonics are obtained by focusing (1 m focal lens) a few mJ of the ‘salle rouge’ laser inside a 5-mm-long gas cell filled with 40 mBar Neon. The harmonic generation signal is then optimized by adjusting the amount of energy and the shape of the beam profile using an iris. Intensities of both fundamental and second harmonic, that have been used for the three configurations presented in our manuscript, are given in the caption of the related figures. To isolate the high harmonics from the fundamental and second harmonic radiations ( ω and 2 ω ), a 400-nm-thick aluminium filter is inserted into the laser path. Generation of the second harmonic The second harmonic is generated by a BBO crystal placed, under vacuum, into the laser path after the focusing lens to obtain a high enough laser fluence for efficient frequency conversion. This crystal has strong negative uniaxial bi-refringence and can be phase-matched for type I in the ‘ooe’ configuration, that is, ω in ordinary polarization yields 2 ω in extraordinary polarization. Due to crystal dispersion effects, the temporal envelops and phases of ω and 2 ω pulses are shifted. This has been calculated with the SNLO (Select Non-Linear Optics) software. The phase shift between the two colours is fixed by the crystal thickness and is ~п/2 for 100-microns-thick BBO crystal as well as for 250 microns. This is evaluated for a perfect condition of phase matching. Detection of the harmonics and measurement of their polarization For evaluating the polarization of different harmonic orders, the spectral components are first separated spatially by a spectrometer. This later is composed of a platinum-coated toroidal mirror (4° grazing incidence angle), which refocus the harmonics, and of a reflective plane grating (120 lines mm −1 , 2.5° grazing incidence angle). A charge-coupled device (CCD) camera ( Fig. 1a ) is used to detect each harmonic order. Upstream of the CCD camera, the harmonic beam is reflected by a [Mo (6.4 nm)/Si (9.6 nm)] × 20 multilayer mirror (45° incidence angle). This mirror acts as an analyser since the ratio between the p and s reflectivities (respectively, R p and R s) is very small at this incidence angle and in the measured spectral range (45° is very close to the Brewster’s angle for each harmonic wavelength). We define the extinction ratio of this analyser as . The multilayer mirror and the CCD camera can be rotated around the optical axis ( θ , Fig. 1a ). The intensity recorded on the camera then follows the Malus’law and can be expressed according to the formula: I = I 0 ( A ( e )*cos (2 θ )+1) where and A ( e ) a function of e (for a perfect analyser A ( e )=1). Figure 2 presents then the evolution of the normalized intensity ; every 20 degrees, each measurement consists in the accumulation of 20,000 shots (20 accumulations of 1 s). The ellipticity of each harmonic in the two-colour configuration is evaluated from equation (1), which will be derived below. First, the ellipticity can be expressed as follows [17] assuming that e is small, which is naturally correct at Brewster’s angle: where and I minor and I major are the intensities on the minor and major axis of the ellipse. as . Then, one can replace e by (I min /I max ) ω , the ratio of intensity measured for harmonics generated only using ω , assuming that the harmonics produced in this case are linearly polarized, which has been demonstrated several times over the past years. An accurate measurement of the s and p reflectivity ratio for the odd orders is performed from 31st to 43rd harmonics using ω as a driving laser. (I min /I max ) ω and consequently e vary from 0.07 to 0.05 respectively, confirming the first approximation ( ). We estimated the response of the system to linear polarization at intermediate wavelengths (corresponding to even orders) not sampled with the linearly polarized harmonics (only odd harmonics are generated) as the average of the two surrounding odd-order ratios. Finally, the grating, as any other optical component, affects the polarization of the beam. However, this effect is very small due to the grazing incidence configuration. This has been measured precisely by fitting the data of ref. 22 obtained in the same optical configuration. For example, for the 43rd harmonic the dephasing between s and p components of the polarization Δ ϕ ~0° and R P /R s ~0.95, and for the 45th harmonic Δ ϕ ~0° and R P /R s ~1. X-ray magnetic circular dichroism We measured the XMCD of a 50-nm-thick Ni film deposited on a 70 nm Si 3 N 4 membrane and capped with 3 nm of Al. This sample is placed in the middle of an assembly consisting of four permanent magnets generating an out-of-plane magnetic field of 0.5 T at the sample position, which induced an out-of-plane magnetization in the Ni film. The whole set-up, the assembly generating this field and the sample, can be rotated together. Thus, the magnitude of the magnetization projection on the optical axis is exactly the same for positive and negative fields. We recorded alternatively the transmitted harmonics spectrum (using 4,960 lines mm −1 reflective plane grating from Horiba Jobin Yvon company at 15° grazing incidence angle) for the two opposite directions (labelled +and −) of the Ni film magnetization along the beam axis. In total, for each direction, 20 accumulations of 30,000 pulses were performed. The XMCD signal is given by: where I + and I − are the transmitted intensities of the harmonics for the two opposite magnetizations of Ni. This signal is then normalized by the one obtained for linearly polarized harmonics ( ω only) for which the XMCD vanishes. This allows us to correct the signal for imperfect alignment of the set-up and non-symmetry on the sample (aluminium on one side and silicon nitride on the other). In addition, to get rid of possible variations of the laser intensity, we shifted the even harmonics signal (the most sensitive order type to laser intensity variation) to the odd harmonics signal. Indeed, such intensity variation can cause a variation of I ω / I 2ω and then subsequently a change of the ratio between odd and even harmonic amplitudes inside the spectrum, creating finally a fake difference of the XMCD traces between both order types. These effects can arise in the spectral ranges for which the XMCD effect is weak. This, in return, prevents from determining whether an asymmetry of the XMCD effect, located particularly in the 60–65 eV range, or a helicity change of the source are existing or not in these spectral regions. How to cite this article: Lambert, G. et al . Towards enabling femtosecond helicity-dependant spectroscopy with high-harmonic sources. Nat. Commun. 6:6167 doi: 10.1038/ncomms7167 (2015).